Steric hindrance between S4 and S5 of the KCNQ1/KCNE1 channel hampers pore opening In voltage-gated K + channels, membrane depolarization induces an upward movement of the voltage-sensing domains (VSD) that triggers pore opening. KCNQ1 is a voltage-gated K + channel and its gating behaviour is substantially modulated by auxiliary subunit KCNE proteins. KCNE1, for example, markedly shifts the voltage dependence of KCNQ1 towards the positive direction and slows down the activation kinetics. Here we identify two phenylalanine residues on KCNQ1, Phe232 on S4 (VSD) and Phe279 on S5 (pore domain) to be responsible for the gating modulation by KCNE1. Phe232 collides with Phe279 during the course of the VSD movement and hinders KCNQ1 channel from opening in the presence of KCNE1. This steric hindrance caused by the bulky amino-acid residues destabilizes the open state and thus shifts the voltage dependence of KCNQ1/KCNE1 channel. Voltage-gated ion channels are activated by membrane potential and contribute to electrical activity in many excitable tissues. They have a tetrameric structure (or pseudotetrameric structure in Na + and Ca 2+ channels), which consists of four six-transmembrane subunits [1] , [2] . The first four transmembrane segments (S1–S4) compose a voltage-sensing domain (VSD), which senses the membrane potential by positively charged amino-acid residues (arginine or lysine) on the S4 segment, the essential part of the voltage sensor. The latter two transmembrane segments (S5–S6) compose a pore domain (PD), which contains a selectivity filter and a gate for the flow of ions. One voltage-gated ion channel contains a single tetrameric PD surrounded by four isolated VSDs [3] . When the membrane potential is depolarized, the four VSDs move from the down (resting) state to the up (activated) state independently, and after all four VSDs reach the upstate, the channel proceeds to the concerted final opening step [4] . KCNQ1 encodes a voltage-gated potassium channel α-subunit. KCNQ1 is widely expressed in various tissues including the heart, where a genetic abnormality in KCNQ1 is known to cause long QT syndrome, a type of cardiac arrhythmia [5] , [6] . Although the KCNQ1 tetramer forms a functional ion channel like other voltage-gated potassium channels, the gating of KCNQ1 may not require all VSDs to be in the upstate for opening, unlike most of the other voltage-gated potassium channels [7] , [8] , [9] . On the other hand, KCNQ1 can have KCNE1 as an auxiliary subunit [10] , [11] . Up to four (or two) KCNE1 subunits bind to the KCNQ1 channel [12] , [13] , [14] , [15] , [16] , [17] and dramatically change various KCNQ1 channel properties including activation/deactivation kinetics, voltage dependence and single channel conductance [10] , [11] , [18] , [19] , [20] . As the slowly activating KCNQ1/KCNE1 channel (also known as the I Ks channel in the heart) plays a particularly critical role in controlling cardiac excitability, how KCNE1 modulates the gating of KCNQ1 has been one of the central questions in the field. KCNE1 has been reported to bind to the PD of KCNQ1 [21] , [22] , but growing evidence suggests the possibility that the VSD could be an interaction site as well [23] , [24] , [25] , [26] . By using the substituted cysteine accessibility method (SCAM) [27] , [28] , two groups including ours previously showed that KCNE1 slows the reaction rate of extracellular MTS reagents with the S4 segment, indicating that KCNE1 stabilizes the downstate of the VSD [23] , [29] . Other site-directed mutagenesis studies also suggest that KCNE1 changes the VSD movement or conformation [30] , [31] , [32] , [33] . In addition, recent voltage clamp fluorometry (VCF) experiments clearly showed that KCNE1 alters VSD movement [34] , [35] . Based on these evidences, it is reasonable to think that KCNE1 slows the gating of KCNQ1, if not exclusively, via the VSD. However, it is still largely unknown how KCNE1 changes the VSD movement and gating. Here we identify two phenylalanine residues, Phe232 on the S4 segment and Phe279 on the S5 segment, as key players in shifting the voltage dependence in the presence of KCNE1. Both amino-acid residues showed side-chain volume-dependent shift of conductance–voltage ( G – V ) relationship only in the presence of KCNE1, suggesting that Phe232 and Phe279 are involved in the opening of KCNQ1/KCNE1 channel. To examine if these two phenylalanine residues are important for the gating of KCNQ1/KCNE1 channel, we applied VCF to compare the S4 movement and the ionic current simultaneously. The S4 movement and the ionic current were almost synchronized in the phenylalanine mutants while there was a substantial delay between the S4 movement and the ionic current in the wild-type (WT) KCNQ1/KCNE1 channel. This supports the initial notion that Phe232 and Phe279 are involved in the opening in the presence of KCNE1. Our present data suggests that steric hindrance of Phe232 and Phe279 destabilize the open state, and thus make KCNQ1/KCNE1 channel harder to be activated. Side-chain volume at Phe232 on S4 correlates with G – V curve KCNE1 shifts the conductance–voltage ( G – V ) relationship of the KCNQ1 channel in the positive direction ( Fig. 1a ). We previously made a series of cysteine mutants of the S4 segment for experiments of the SCAM [23] . While we eventually picked A226C mutant for the SCAM, we initially noticed that the F232C mutant lacked the characteristic positive G – V shift induced by KCNE1. The G – V shift induced by KCNE1 for KCNQ1 WT was +29 mV (from −20 to +9 mV); on the other hand, the F232A mutant showed a rather negative G – V shift of −4 mV (from −16 to −20 mV) ( Fig. 1a ). 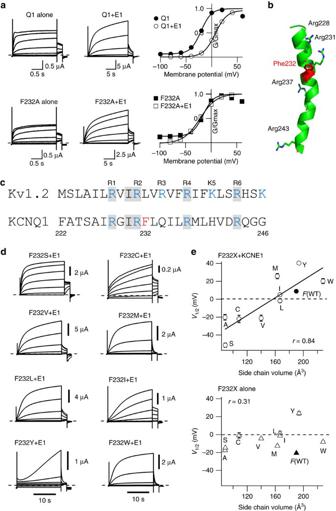Figure 1: Side-chain volume of Phe232 in S4 correlates with theG–Vrelationships in the presence of KCNE1. (a) Current traces under two-electrode voltage clamp andG–Vcurves for WT KCNQ1 and F232A mutant in the absence and the presence of KCNE1 inXenopusoocytes. Currents were elicited by stepping membrane voltage from the −90 mV holding potential to between −100 and +60 mV for 2 s (KCNQ1 current) or between −80 and +40 mV for 20 s (KCNQ1+KCNE1 current). The time scale is 10 times longer in the presence of KCNE1. Dotted lines indicate zero current level.G/Gmax, which is normalized tail current amplitude, was plotted against membrane potential for presentation of the G–Vcurves.G–Vcurves were fitted with a Boltzmann function (equation (1) in Methods). (b) Structure of the S4 segment of the KCNQ1 open-state model37. Phe232 is coloured in red. Side chains of Phe232 and four Arg residues are depicted. (c) Alignment of amino-acid sequence of the S4 segments of Kv1.2 and KCNQ1. Conserved amino-acid residues are shaded in grey. Positively charged amino-acid residues are coloured in blue. Phe232 is coloured in red. (d) Ionic currents for Phe232 mutants with KCNE1. (e)V1/2values of theG–Vcurves are plotted against the side-chain volume for each F232X mutant in the presence (upper) and absence (bottom) of KCNE1. Data are mean±s.e.m.;n=3–47 (Supplementary Table 1). Dotted line indicates 0 mV. Correlation coefficients are 0.84 and 0.31, respectively. The linear regression is shown as a straight line. Filled data points are from the WT and open data points are from the mutants. Although KCNE1 failed to shift the G – V curve of F232A, KCNE1 increased the current amplitude of F232A by 4.7-fold (6.7-fold increase in KCNQ1 WT) ( Supplementary Table 1 ). Phe232 is located between the second arginine ‘R2’ (Arg231) and the fourth arginine ‘R4’ (Arg237) on the S4 segment (‘R3’ is glutamine in KCNQ1, though). Phe232 is not conserved in potassium channels other than the KCNQ family ( Fig. 1b,c ). Figure 1: Side-chain volume of Phe232 in S4 correlates with the G – V relationships in the presence of KCNE1. ( a ) Current traces under two-electrode voltage clamp and G – V curves for WT KCNQ1 and F232A mutant in the absence and the presence of KCNE1 in Xenopus oocytes. Currents were elicited by stepping membrane voltage from the −90 mV holding potential to between −100 and +60 mV for 2 s (KCNQ1 current) or between −80 and +40 mV for 20 s (KCNQ1+KCNE1 current). The time scale is 10 times longer in the presence of KCNE1. Dotted lines indicate zero current level. G / G max , which is normalized tail current amplitude, was plotted against membrane potential for presentation of the G– V curves. G – V curves were fitted with a Boltzmann function (equation (1) in Methods). ( b ) Structure of the S4 segment of the KCNQ1 open-state model [37] . Phe232 is coloured in red. Side chains of Phe232 and four Arg residues are depicted. ( c ) Alignment of amino-acid sequence of the S4 segments of Kv1.2 and KCNQ1. Conserved amino-acid residues are shaded in grey. Positively charged amino-acid residues are coloured in blue. Phe232 is coloured in red. ( d ) Ionic currents for Phe232 mutants with KCNE1. ( e ) V 1/2 values of the G – V curves are plotted against the side-chain volume for each F232X mutant in the presence (upper) and absence (bottom) of KCNE1. Data are mean±s.e.m. ; n =3–47 ( Supplementary Table 1 ). Dotted line indicates 0 mV. Correlation coefficients are 0.84 and 0.31, respectively. The linear regression is shown as a straight line. Filled data points are from the WT and open data points are from the mutants. Full size image To understand the mechanism how Phe232 plays a role in the G – V shift by KCNE1, we mutated Phe232 to various amino-acid residues including S, V, M, L, I, Y, W. All of them were expressed well both with and without KCNE1 ( Fig. 1d and Supplementary Table 1 ). Interestingly, midpoint of the G – V curve ( V 1/2 ) showed a positive correlation with side-chain volume, only in the presence of KCNE1 ( Fig. 1e ). In the presence of KCNE1, V 1/2 of WT KCNQ1 was +9±1 mV ( n =47), F232A and F232S, the smallest amino-acid residues among them, showed −20±3 ( n =16) and −51±2 mV ( n =6), respectively, and the largest F232W showed +20±3 mV ( n =9). A correlation coefficient ( r ) between the V 1/2 and side-chain volume is 0.84, indicating that the equilibrium of open and closed states is strongly correlated with the side-chain bulkiness of Phe232 on the S4 segment in the presence of KCNE1. The slope of the linear regression was 0.49 mV Å −3 ( Fig. 1e ). Chowdhury et al . [36] recently showed that gating analysis using Boltzmann equation from macroscopic currents is not necessarily accurate, mainly because the channel activation process cannot be always simplified as a two-state model assumed in the analysis. Keeping this point in mind as an alert, we still continued to apply Boltzmann analysis for mutant evaluation because it is a convenient way to grasp the tendency of the effects of mutations. Side-chain volume at Phe279 on S5 correlates with G – V curve If the bulkiness of Phe232 determines V 1/2 with KCNE1, Phe232 may physically collide with another amino-acid residue during the course of transition from the downstate to the upstate in the presence of KCNE1. If such an opponent exists, it may also show a side-chain volume-dependent V 1/2 change in the presence of KCNE1. According to the structural models for KCNQ1, Phe232 faces the S5 segment both in the closed and open states [37] . Phe232 is in proximity to Ile274 in the closed-state model and close to Phe279 in the open-state model ( Fig. 2a ). Generally, the S4 segment of the voltage-gated ion channel rotates and moves upward (towards extracellular side) upon depolarization. Phe232 on the S4 segment probably moves upward, rotates clockwise (from the extracellular side) and passes through Phe279 when the membrane is depolarized ( Fig. 2a ). We therefore hypothesized that the bulky amino-acid residue on the S5 segment might be an obstacle for Phe232. The S5 segment of KCNQ1 contains three phenylalanine residues (Phe270, Phe275 and Phe279), and we mutated all of them to alanine residues ( Fig. 2b ). Besides them, Ile274, which is known as a site of the short QT syndrome, was also mutated to alanine and valine (I274V, the same mutant found in the patient) [38] , [39] . Among these mutants, I274A (−7±3 mV, n =15), I274V (−12±3 mV, n =12) and F279A (−38±5 mV, n =12) showed negative V 1/2 values in the presence of KCNE1 ( Fig. 2c,d ). 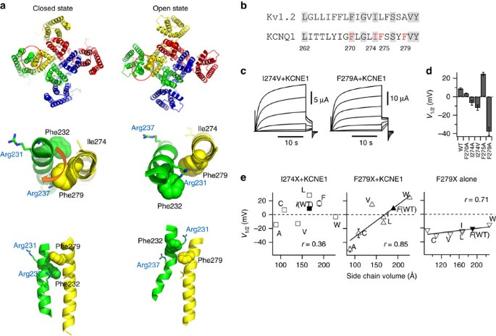Figure 2: Side-chain volume of Phe279 in S5 correlates with theG–Vrelationships in the presence of KCNE1. (a) (top) Top views of the KCNQ1 tetramer in the closed state and the open state. Each subunit is coloured differently, and one of the S4–S5 pairs is circled in red. (middle) Top views of the S4 (green) and S5 (yellow) segments in the closed-state and the open-state KCNQ1 models. The structural models are slightly tilted to show the spatial relationships of Phe232 and Phe279. Side chains of Phe232 and Phe279 are depicted as spheres and side chains of Arg231, Arg237 and Ile274 are depicted as sticks. Upward and rotating movement of S4 during depolarization is illustrated as an orange arrow in the closed-state model. (bottom) Side views of the S4 (green) and S5 (yellow) segments in the closed-state and the open-state KCNQ1 model. (b) Alignment of the amino-acid sequence of the S5 segments of Kv1.2 and KCNQ1. Conserved amino-acid residues are shaded in grey. Mutated residues in this study are coloured in red. (c) Current traces of I274V+KCNE1 and F279A+KCNE1. Currents were elicited by stepping membrane voltage from the −90 mV holding potential to between −100 and +40 mV. (d)V1/2values for WT and the S5 mutants with KCNE1 are plotted. Data are mean±s.e.m.;n=2–15 (Supplementary Table 1). (e)V1/2side-chain volume relationships for I274X mutants with KCNE1 (left), F279X mutants with KCNE1 (middle) and F279X without KCNE1 (right). Data are mean±s.e.m.;n=4–15 (Supplementary Table 1). Correlation coefficients are 0.36, 0.85 and 0.71, respectively. Straight lines indicate linear regressions. Filled data points are from the WT and open data points are from the mutants. Figure 2: Side-chain volume of Phe279 in S5 correlates with the G – V relationships in the presence of KCNE1. ( a ) (top) Top views of the KCNQ1 tetramer in the closed state and the open state. Each subunit is coloured differently, and one of the S4–S5 pairs is circled in red. (middle) Top views of the S4 (green) and S5 (yellow) segments in the closed-state and the open-state KCNQ1 models. The structural models are slightly tilted to show the spatial relationships of Phe232 and Phe279. Side chains of Phe232 and Phe279 are depicted as spheres and side chains of Arg231, Arg237 and Ile274 are depicted as sticks. Upward and rotating movement of S4 during depolarization is illustrated as an orange arrow in the closed-state model. (bottom) Side views of the S4 (green) and S5 (yellow) segments in the closed-state and the open-state KCNQ1 model. ( b ) Alignment of the amino-acid sequence of the S5 segments of Kv1.2 and KCNQ1. Conserved amino-acid residues are shaded in grey. Mutated residues in this study are coloured in red. ( c ) Current traces of I274V+KCNE1 and F279A+KCNE1. Currents were elicited by stepping membrane voltage from the −90 mV holding potential to between −100 and +40 mV. ( d ) V 1/2 values for WT and the S5 mutants with KCNE1 are plotted. Data are mean±s.e.m. ; n =2–15 ( Supplementary Table 1 ). ( e ) V 1/2 side-chain volume relationships for I274X mutants with KCNE1 (left), F279X mutants with KCNE1 (middle) and F279X without KCNE1 (right). Data are mean±s.e.m. ; n =4–15 ( Supplementary Table 1 ). Correlation coefficients are 0.36, 0.85 and 0.71, respectively. Straight lines indicate linear regressions. Filled data points are from the WT and open data points are from the mutants. Full size image We subsequently mutated Ile274 and Phe279 to various other amino-acid residues to test the volume dependence of V 1/2 as seen in Phe232 mutants in the presence of KCNE1 ( Fig. 2e and Supplementary Fig. 1 ). Ile274 mutants with KCNE1 did not show a clear volume-dependent V 1/2 change ( r =0.36) ( Fig. 2e left and Supplementary Fig. 1a ). Therefore, Ile274 may not be a collision site for Phe232 although they may be in a close proximity in the closed-state model ( Fig. 2a ). Phe279, on the other hand, showed a clear side-chain volume dependence in the presence of KCNE1 ( r =0.85) ( Fig. 2e middle and Supplementary Fig. 1b ). The slope of the linear regression was 0.46 mV Å −3 , which is comparable to the slope of F232X+E1 (0.49 mV Å −3 ; Fig. 1e ). A high correlation efficient between V 1/2 and side-chain volume was also seen in the absence of KCNE1 ( r =0.71; Fig. 2e right and Supplementary Fig. 1c ); however, the slope of the linear regression was almost six times shallower in the absence of KCNE1 (0.08 mV Å −3 ; Fig. 2e ), indicating that side-chain volume dependence is weak in the absence of KCNE1. Taken together, the bulky side chain of Phe279 on the S5 segment also defines the energy difference between the closed and open states in the presence of KCNE1. Functional and steric interaction between Phe232 and Phe279 As Phe232 and Phe279 mutants showed a similar side-chain volume-dependent V 1/2 change, we predicted that Phe232 and Phe279 are functionally coupled. To examine this idea, we made a double mutant of F232A and F279A ( Supplementary Fig. 2a ). The V 1/2 of F232A/F279A with KCNE1 was −25±1 mV (mean±s.e.m. ; n =5), which is even more positive than the V 1/2 of F279A single mutant (−38±5 mV, n =12) ( Supplementary Fig. 2b ), indicating mutation effects of F232A and F279A are not additive. This non-additivity of F232A and F279A suggests that these phenylalanine residues are functionally coupled. If Phe232 collide with Phe279 during activation as we hypothesized, these residues should be not only functionally coupled but also in close proximity at a certain point of the transition from the downstate to the upstate of the S4 segment. To test this idea, we made a double mutant of F232C/F279C and examined disulphide formation between the two introduced cysteine residues. We applied a pair of sets of depolarizing pulses from −80 mV to +40 mV to F232C/F279C+KCNE1, and −100 mV to +60 mV to F232C/F279C alone ( Fig. 3a,b , inset). In the presence of KCNE1, F232C/F279C showed larger instantaneous current and a constitutively active component during the second set of pulses ( Fig. 3a ). This suggests that F232C and F279C spontaneously formed a disulphide bond during depolarization and made the channel constitutively active at least partially. A similar result was also observed in the absence of KCNE1 ( Fig. 3b ). This result was somewhat unexpected because both Phe232 and Phe279 mutants showed a minor or no side-chain volume dependence in the absence of KCNE1 (see Figs 1e , 2e ). The distance between Phe232 and Phe279 becomes short during depolarization regardless of the presence of KCNE1. This result is consistent with the KCNQ1 structural models (see Fig. 2a ) [37] . 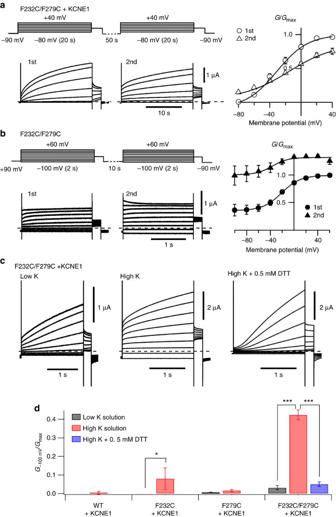Figure 3: Disulphide bond formation between F232C and F279C. (a) Current traces and theG–Vrelationships of F232C/F279C with KCNE1 for the first and second sets of depolarization. Data (average±s.e.m;n=3) are normalized byGmaxof the first set. Currents were elicited from the −90 mV holding potential to between −80 mV and +40 mV for 20 s with a 50-s interval between the start of each depolarization. After the end of the first set, we waited for 50 s before the start of the second set (inset).G–Vcurves are fitted with a Boltzmann function. (b) Current traces and theG–Vrelationships of F232C/F279C without KCNE1 for the first and second sets of depolarization. Data (average±s.e.m;n=3) are normalized byGmaxof the first set. Currents were elicited from the −90 mV holding potential to between −100 and +60 mV for 2 s with a 10-s interval between the start of each depolarization. After the end of the first set, we waited for 10 s before the start of the second set (inset).G–Vcurves are fitted with a Boltzmann function. Number of experiments is 3. (c) Representative current traces of F232C/F279C+KCNE1 after 3 h incubation in low K, high K and high K with 0.5 mM DTT. Oocytes in high K solution were back to low K solution at least for 3 min before recording to relieve accumulated open-state channel without a disulphide bond formation. Currents were elicited from the −90 mV holding potential to between −100 and +60 mV for 2 s. (d) Constitutively active components (ratio of conductance at −100 mV (G−100 mV) and maximum conductance (Gmax)) were plotted. Statistical significance were evaluated by Tukey–Kramer test (n=4–9). Figure 3: Disulphide bond formation between F232C and F279C. ( a ) Current traces and the G – V relationships of F232C/F279C with KCNE1 for the first and second sets of depolarization. Data (average±s.e.m; n =3) are normalized by G max of the first set. Currents were elicited from the −90 mV holding potential to between −80 mV and +40 mV for 20 s with a 50-s interval between the start of each depolarization. After the end of the first set, we waited for 50 s before the start of the second set (inset). G – V curves are fitted with a Boltzmann function. ( b ) Current traces and the G–V relationships of F232C/F279C without KCNE1 for the first and second sets of depolarization. Data (average±s.e.m; n =3) are normalized by G max of the first set. Currents were elicited from the −90 mV holding potential to between −100 and +60 mV for 2 s with a 10-s interval between the start of each depolarization. After the end of the first set, we waited for 10 s before the start of the second set (inset). G–V curves are fitted with a Boltzmann function. Number of experiments is 3. ( c ) Representative current traces of F232C/F279C+KCNE1 after 3 h incubation in low K, high K and high K with 0.5 mM DTT. Oocytes in high K solution were back to low K solution at least for 3 min before recording to relieve accumulated open-state channel without a disulphide bond formation. Currents were elicited from the −90 mV holding potential to between −100 and +60 mV for 2 s. ( d ) Constitutively active components (ratio of conductance at −100 mV ( G −100 mV ) and maximum conductance ( G max )) were plotted. Statistical significance were evaluated by Tukey–Kramer test ( n =4–9). Full size image We also tested the validity of the disulphide bond formation in WT, F232C, F279C and F232C/F279C with KCNE1 by incubating in low K (2 mM K + ) and high K (98 mM K + ) for 3 h. F232C/F279C with KCNE1 showed high constitutively active component ( G −100 mV / G max ) ( Fig. 3c,d ). This constitutively active component was not seen when 0.5 mM DTT was included in the high K solution ( Fig. 3c,d ). VCF of the Phe mutants If Phe232 and Phe279 mutations truly change V 1/2 or the voltage sensor equilibrium, the voltage sensor movement might be changed in F232A and F279A mutants. We, therefore, applied VCF to directly track the voltage sensor movement in these mutants with simultaneous current recording [34] , [35] , [40] . KCNQ1 with C214A/G219C/C331A mutations (which will be described as WT henceforth), the exactly same construct reported by Osteen et al . [34] , was used as a background. In this construct, two endogenous cysteine residues, one located in the upper part of the S3 (Cys214) and the other located in the upper part of the S6 (C331), have been replaced with alanine to exclusively attach Alexa488 maleimide to G219C on the S3-S4 linker [34] . Neither these mutations nor the introduction of Alexa488 significantly affect the channel properties [34] . In the absence of KCNE1, WT construct showed fluorescence signal mostly when the ionic current was also evoked ( Fig. 4 ). On the other hand, as previously reported [34] , WT with KCNE1 showed a large fluorescence change at hyperpolarized potentials far below the threshold of the ionic current (−40 mV) and did not saturate either end of the voltage (between −160 and +80 mV). The F–V relationship obviously has two components; the first and left-shifted component relative to G - V curve and the 2nd component activating at depolarized potential and seemingly related to channel opening ( G–V relationship) as previously reported by Osteen et al [34] , and as very recently clearly shown by Barro-Soria et al . [41] F – V relationships of F232A+KCNE1 and F279A+KCNE1 are basically similar to that of WT, having the two fluorescent components. However, the second components are larger in the Phe mutants, especially in F279A+KCNE1, probably due to the left-shifted G – V curves in the mutants if the second component actually tracks the channel opening as suggested [34] . 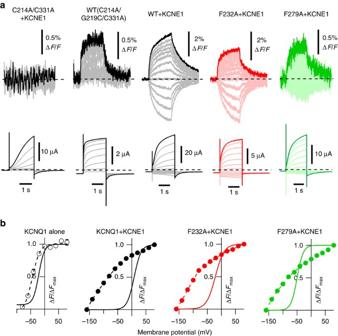Figure 4: Fluorescence–voltage relationships for KCNQ1 and the Phe mutants. (a) Fluorescence traces (upper row) and ionic currents (bottom row) for C214A/C331A+KCNE1 (negative control), KCNQ1 WT (C214A/G219C/C331A) alone, WT+KCNE1, F232A+KCNE1 (red) and F279A+KCNE1 (green) attached with Alexa488 maleimide are shown. Only fluorescent and current traces at the highest membrane potential are in dark colour for clarity. Dashed lines indicate the zero level for fluorescence and current. Oocytes were stimulated by stepping membrane voltage from the −80 mV holding potential to between −160 and +80 mV. Fluorescence was decreased by hyperpolarization and increased by depolarization. Fluorescence reduction due to photobleaching was compensated by the equation (2) described in Methods. (b) ΔF–Vrelationships for WT and each mutant with KCNE1 are shown. Normalized ΔFvalues for WT (open black circles;n=4) WT+KCNE1 (filled black circles;n=10), F232A+KCNE1 (filled red circles;n=3) and F279A+KCNE1 (filled green circles;n=3) are plotted.G-Vrelationships fromFigs 1,2are also plotted for comparison (solid curves). Figure 4: Fluorescence–voltage relationships for KCNQ1 and the Phe mutants. ( a ) Fluorescence traces (upper row) and ionic currents (bottom row) for C214A/C331A+KCNE1 (negative control), KCNQ1 WT (C214A/G219C/C331A) alone, WT+KCNE1, F232A+KCNE1 (red) and F279A+KCNE1 (green) attached with Alexa488 maleimide are shown. Only fluorescent and current traces at the highest membrane potential are in dark colour for clarity. Dashed lines indicate the zero level for fluorescence and current. Oocytes were stimulated by stepping membrane voltage from the −80 mV holding potential to between −160 and +80 mV. Fluorescence was decreased by hyperpolarization and increased by depolarization. Fluorescence reduction due to photobleaching was compensated by the equation (2) described in Methods. ( b ) Δ F – V relationships for WT and each mutant with KCNE1 are shown. Normalized Δ F values for WT (open black circles; n =4) WT+KCNE1 (filled black circles; n =10), F232A+KCNE1 (filled red circles; n =3) and F279A+KCNE1 (filled green circles; n =3) are plotted. G - V relationships from Figs 1 , 2 are also plotted for comparison (solid curves). Full size image We next evaluated the kinetics of voltage sensor movement. The rising phase of fluorescence could be fitted with either a single or double exponential function ( Fig. 5a ). In WT+KCNE1, the (faster) time constant started around 1 s and voltage dependently decreased to below 0.1 s. A slower time constant emerged from −20 mV, and was ~1 s with less voltage dependence ( Fig. 5b ). Interestingly, WT without KCNE1 showed virtually the same time constants as those of WT+KCNE1 ( Fig. 5a,b ). However, the ratio of the slow and fast components is clearly different and the slow component is dominant in WT+KCNE1 ( Fig. 5c ). Faster time constants of F232A+KCNE1 tended to be faster than those of WT at any membrane potential, although statistical significance was confirmed only at −80 and −20 mV. On the other hand, faster time constants were slightly slower in F279A+KCNE1 than those of WT+KCNE1 ( Fig. 5a,b ). Slower time constants and the amplitude of slower component were not significantly different among WT and the two F-A mutants ( Fig. 5b,c ). In summary, the kinetics of VCF of F232A+KCNE1 and F279A+KCNE1 are not largely different from that of WT+KCNE1. The rising kinetics of the S4 voltage sensor movement does not explain why F232A+KCNE1 and F279A+KCNE1 showed negative V 1/2 than WT+KCNE1 in the previous experiments. 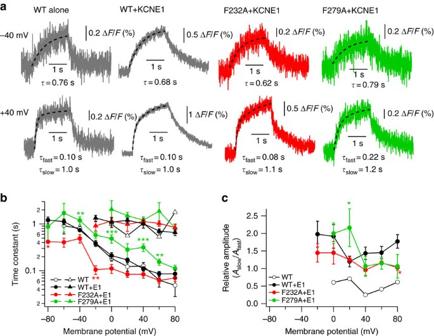Figure 5: Kinetics of the S4 segment movement upon depolarization are not changed by the Phe mutations. (a) VCF recording traces for WT, WT+KCNE1 (grey), F232A+KCNE1 (red) and F279A+KCNE1 (green) by depolarization at −40 and +40 mV. Dotted lines are the fitting by a single exponential function for traces elicited by −40 mV depolarization, and by a double exponential function for traces by +40 mV. Time constants deduced from fitting are shown below. (b) Fast (circles) and slow (triangles) time constants for the fluorescence rises for WT (n=4), WT+KCNE1 (n=16), F232A+KCNE1 (n=7) and F279A+KCNE1 (n=6) are plotted against membrane potential. (c) The relative amplitude of the fast and slow components is plotted against membrane potential. Figure 5: Kinetics of the S4 segment movement upon depolarization are not changed by the Phe mutations. ( a ) VCF recording traces for WT, WT+KCNE1 (grey), F232A+KCNE1 (red) and F279A+KCNE1 (green) by depolarization at −40 and +40 mV. Dotted lines are the fitting by a single exponential function for traces elicited by −40 mV depolarization, and by a double exponential function for traces by +40 mV. Time constants deduced from fitting are shown below. ( b ) Fast (circles) and slow (triangles) time constants for the fluorescence rises for WT ( n =4), WT+KCNE1 ( n =16), F232A+KCNE1 ( n =7) and F279A+KCNE1 ( n =6) are plotted against membrane potential. ( c ) The relative amplitude of the fast and slow components is plotted against membrane potential. Full size image S4 movement and gating are synchronized in the Phe mutants We next compared the kinetics of the VCF and simultaneously recorded ionic current ( Fig. 6a ). In WT KCNQ1 without KCNE1, the ionic current and the fluorescence intensity almost completely overlapped ( Fig. 6a first row and 6b upper left), as previously reported [9] , [34] . In WT KCNQ1+KCNE1, on the other hand, the fluorescence signal always preceded the ionic current. At −40 mV, where virtually no current was seen in the KCNQ1/KCNE1 channel, a clear fluorescence signal was already observed. The ionic current started to be seen from −20 mV, and the fluorescence signal preceded the ionic current, which showed characteristic sigmoidal delay ( Fig. 6a second row). Faster time constants of the ionic current overlapped somewhat with the slower time constants of the VCF signal ( Fig. 6b , upper right). Therefore, even though the time constants of fast and slow components of the KCNQ1 S4 movement by VCF were virtually the same in the absence and presence of KCNE1 (see in Fig. 5 ), there was a substantial delay of current activation after the S4 movement in the KCNQ1/KCNE1 channels. In F279A+KCNE1, the VCF signal and ionic current were quite well synchronized ( Fig. 6a , fourth row). In F279A+KCNE1, faster time constants of the VCF signals and ionic currents were very close at any voltage where current was detected (from −60 to +80 mV) ( Fig. 6b bottom right). F232A+KCNE1 showed an intermediate phenotype of the WT KCNQ1+KCNE1 and F279A+KCNE1: the fluorescence signal slightly preceded the ionic current ( Fig. 6a third row), and the faster activation time constants sit between fast and slow time constants of the VCF signal ( Fig. 6b bottom left). Therefore, Phe279 and probably Phe232 play a significant role in coupling (decoupling) the S4 sensor movement and pore opening in the presence of KCNE1 rather than changing the S4 sensor movement. 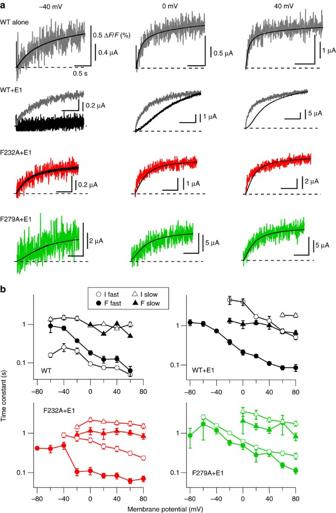Figure 6: Current activation and fluorescence rise overlap in the Phe mutants. (a) Ionic currents (black traces) and fluorescence traces (grey traces) for WT and WT+KCNE1, red traces for F232A+KCNE1 and green traces for F279A+KCNE1) at −40, 0, +40 mV are superimposed. Left vertical bars and horizontal bars indicate 0.5 ΔF/F% and 0.5 s, respectively. (b) Fast (circles) and slow (triangles) time constants for ionic currents (open symbols) and fluorescence changes (filled symbols) are compared. Figure 6: Current activation and fluorescence rise overlap in the Phe mutants. ( a ) Ionic currents (black traces) and fluorescence traces (grey traces) for WT and WT+KCNE1, red traces for F232A+KCNE1 and green traces for F279A+KCNE1) at −40, 0, +40 mV are superimposed. Left vertical bars and horizontal bars indicate 0.5 Δ F / F % and 0.5 s, respectively. ( b ) Fast (circles) and slow (triangles) time constants for ionic currents (open symbols) and fluorescence changes (filled symbols) are compared. Full size image In this study, we identified Phe232 in the S4 segment and Phe279 in the S5 segment as molecular determinants for the G – V relationship in the KCNQ1/KCNE1 channel. The S4 segment, which possesses several positively charged amino-acid residues ( Fig. 1b,c ), is the central part of the voltage sensor domain in most of the voltage-gated ion channels. When the membrane potential is depolarized, the S4 segment rotates and moves up towards the extracellular side, and that eventually leads to the opening of the PD [1] , [42] . Phe232 is located next to the second arginine Arg231 and rotates and moves upward along with the S4 segment during depolarization ( Fig. 2a ). The side-chain volume-dependent V 1/2 changes in F232X mutants +KCNE1 suggested that a bulky phenylalanine side chain on the S4 segment could be a hindrance and might collide with another amino-acid residue during the S4 transition to the upstate. According to the KCNQ1 structural models, Phe232 faces the S5 segment both in the closed and open states ( Fig. 2a ) [37] . We next identified Phe279, which is located at the top of the S5 segment, as a putative obstacle for Phe232. Most notably, F279X mutants also showed a side-chain volume-dependent V 1/2 change in the presence of KCNE1 ( Fig. 2e ). This supports the idea that bulky Phe232 and Phe279 are physical obstacles for opening, or simply destabilize the open state ( Fig. 7 ). In the downstate at hyperpolarized potential, Phe232 is located deep in the membrane. When the membrane potential is depolarized, the S4 segment starts to rotate in the clockwise direction and move upward to the pre-upstate. During or after the activation, Phe232 on the S4 segment may collide with Phe279 on the S5 segment and that may destabilize the final upstate and/or prevent the channel from opening ( Fig. 7 , upper row). Therefore, to keep the open state of WT KCNQ1/KCNE1 channel, higher depolarization is required. This final transition from the pre-upstate to the upstate may correspond to the second voltage sensor movement proposed by Barro-Soria [41] , which is seen as the second fluorescent component in Fig. 4a,b . In contrast, F232A+KCNE1 and F279A+KCNE1 have less conflict between S4 and S5 segments. In these cases, the upstate is relatively stable and very high depolarization is not required to enter and stay in the upstate ( Fig. 7 , bottom row). 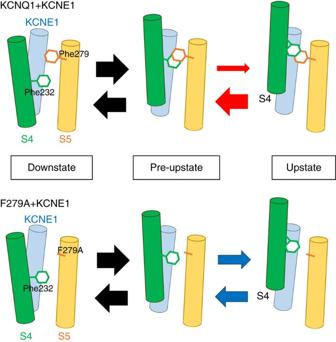Figure 7: Steric hindrance of Phe232 and Phe279 destabilize the upstate. In the presence of KCNE1 (light blue column), Phe232 in the S4 segment (green column) collides with Phe279 in the S5 segment (yellow column) during or after activation. This steric interaction destabilizes upstate, presumably by changing the rate constants (red arrows), and thus prevents the channel pore from opening. In F279A+KCNE1 channel, S4 segment can smoothly move up to the upstate and thus the upstate is more stabilized with different rate constants (blue arrows). The first transition between the downstate and the pre-upstate remains intact in the mutant (black arrows). The location of KCNE1 is tentative. Figure 7: Steric hindrance of Phe232 and Phe279 destabilize the upstate. In the presence of KCNE1 (light blue column), Phe232 in the S4 segment (green column) collides with Phe279 in the S5 segment (yellow column) during or after activation. This steric interaction destabilizes upstate, presumably by changing the rate constants (red arrows), and thus prevents the channel pore from opening. In F279A+KCNE1 channel, S4 segment can smoothly move up to the upstate and thus the upstate is more stabilized with different rate constants (blue arrows). The first transition between the downstate and the pre-upstate remains intact in the mutant (black arrows). The location of KCNE1 is tentative. Full size image On the other hand, F232A+KCNE1 and F279A+KCNE1 still showed two components in F – V relationships ( Fig. 4 ). The S4 movements of F232A+KCNE1 and F279A+KCNE1 are highly similar to that of KCNQ1+KCNE1 channel. As the S4 segment of the mutants significantly moves at hyperpolarized potential as in KCNQ1+KCNE1 channel ( Fig. 4 ), prepulse to hyperpolarized potential is expected to affect the activation kinetics in ionic current (Cole–Moore shift) [34] . Smaller delay in the ionic current in the mutants could be explained by Cole–Moore shift, and if that is the case, delay may be regained by prepulse to more hyperpolarized potential. We examined Cole–Moore shifts in the mutants. Prepulses of −160 mV actually regained delay of activation in F232A+KCNE1 and F279A+KCNE1 although the Cole–Moore shifts looked less obvious than in WT+KCNE1 ( Supplementary Fig. 3 ). While S4 segments of F232A+KCNE1 and F279A+KCNE1 definitely move in hyperpolarized potential as clearly shown in Fig. 4 , smaller delay in the mutants could be due to other reasons, for example, faster transition from the downstate to the pre-upstate. There have been several mutation studies on the S4 segment, mainly focusing on the role of the positively charged residues [30] , [31] , [32] , [33] , [43] . Wu et al . [33] have shown that mutations on the first arginine (R1; Arg228) and the second arginine (R2; Arg231) of the S4 segment destabilize the closed state and mutations on the fourth arginine (R4; Arg237) and the six arginine (R6; Arg243) destabilize the open state. According to their model and the structural model by Smith et al . ( Fig. 2a ), R1 and R2 probably make an electrostatic interaction with Glu160 (E1) in the S2 segment in the closed state (the downstate and the pre-upstate in Fig. 7 ), and R4 may make an electrostatic interaction with E1 in the open state (the upstate in Fig. 7 ) [32] , [33] , [37] . Interestingly, while the R1 and R2 mutants are effective both in the absence and presence of KCNE1, the R4 and R6 mutants are less effective in the presence of KCNE1 (ref. 33 ). As Phe232 and Phe279 destabilize the upstate in the presence of KCNE1, the destabilization effect on the upstate by R4/R6 mutation might be masked. Why Phe232 and Phe279 are effective only in the presence of KCNE1? F232C and F279C can form a disulphide bond during depolarization regardless of the presence/absence of KCNE1 ( Fig. 3 ). This result implies that KCNE1 does not rearrange the distance between Phe232 and Phe279. One possible explanation is that the distance between the S4 and S5 segments may be rather flexible in the absence of KCNE1 and Phe232 can avoid a collision with Phe279 during the course of activation. Wu et al . [33] also reported that V221W and A223W (extracellular side of the S4 segment) mutations destabilize the open state of KCNQ1 channel only in the presence of KCNE1. This indicates that the upper part of S4 segment may be packed in the presence of KCNE1 because perturbation by bulky tryptophan is considered to be only effective in a packed environment for protein. Binding of KCNE1 may reduce the flexibility and lower the mobility [44] , so that Phe232 may have a narrower space to avoid Phe279 during depolarization. KCNE1 is known to bind to the PD [21] , [22] and the voltage sensor domain [23] , [25] . However, the precise location of KCNE1 still remains to be elucidated [26] , [44] , [45] , [46] . Where KCNE1 binds to, and how that makes the two phenylalanine residues change the stability of the upstate would be the next open questions. Osteen et al . [34] previously showed that the fluorescence signal from the KCNQ1/KCNE1 channel with Alexa488 on G219C changes over a wide range of voltage from −180 to +80 mV, and it does not reach a saturation point at either end of the voltage range . The F – V relationship is well negatively shifted compared with the G – V curve (we also confirmed that in Fig. 4 ). This is in sharp contrast to the F – V relationship in the absence of KCNE1, which completely overlaps with G – V relationship [9] , [34] . In terms of kinetics, according to our present data, the KCNQ1 channel showed similar time constants of the VCF signals in the absence and the presence of KCNE1 ( Fig. 5a,b ). The major difference was the larger fraction of slow component in WT+KCNE1 than in WT alone ( Fig. 5c ). This implies that the voltage sensor movement may not be very different at least in the initial step (from the downstate to the pre-upstate in Fig. 6 ), and rather the late step (from the pre-upstate to the upstate) may be mainly affected by KCNE1. VCF data by Ruscic et al . [35] using TMRM attached to V221C look very different from the data by Osteen et al . : the G – V and the F – V are both positively shifted and completely overlapped each other in the presence of KCNE1. Although V221C is located just two amino-acid residues closer to the S4 helix compared with G219C, such a subtle difference might make V221C-TMRM more sensitive to the late S4 conformational change related to the pore opening (from the pre-upstate to the upstate in Fig. 7 ) rather than the initial transition (from the downstate to the pre-upstate in Fig. 7 ), which might be sensitively detected by G219C-Alexa488. It would be interesting to see how the fluorescence signal from V221C/F279A (or F232A) +KCNE1 behaves. Our attempts so far have failed because signals from the mutants were too small to be detected. In conclusion, our study demonstrates Phe232 on the S4 and Phe279 on the S5 destabilize the upstate (open state) of KCNQ1 channel only in the presence of KCNE1. Although the detail molecular mechanism how KCNE1 interacts with KCNQ1 channel and modulates KCNQ1 gating still remains to be elucidated, our findings presented here are, at least, part of the whole picture of the unique gating of KCNQ1/KCNE1 channel. Site-directed mutagenesis and electrophysiological recording The cDNA clones of human KCNQ1 in pSP64 vector were subcloned into the SmaI and BamHI sites of pGEMHE vector. The cDNA clone of human KCNE1 in pcDNA3.1 vector was amplified with a T7 primer and a reverse primer (5′-tttaagcttcatggggaaggcttcgtctcagg-3′) to introduce a HindIII site just after the stop codon and subsequently subcloned into the EcoRI and HindIII sites of pGEMHE vector. Site-directed mutagenesis was done by a PCR-based method with KOD Plus (Toyobo). F232A was, for example, separately amplified in two parts: the first part was amplified with a T7 primer and a phosphorylated reverse primer (5′-gcggatgcccctgatggc-3′) and the second part was amplified with a phosphorylated forward primer including F232A mutation (5′-gccctgcagatcctgaggatg-3′) and a reverse primer containing pGEMHE sequence (5′-agcttagagactccattcgg-3′) using the human KCNQ1 pGEMHE construct as a template. The two PCR fragments were then ligated at the phosphorylated blunt ends and subcloned into the KpnI and HindIII sites of pGEMHE vector. Sequences of the primers used in this study are provided in Supplementary Table 2 . The plasmid sequences were confirmed by DNA sequencing. The cRNAs were synthesized with mMESSAGE mMACHINE T7 kit (Life Technologies) from the linearized plasmid cDNA. Xenopus oocytes were collected from frogs anesthetized in water containing 0.15% tricaine. The isolated oocytes were treated with collagenase (2 mg ml −1 ; type 1; Sigma-Aldrich) for 6–7 h to completely remove the follicular cell layer. Oocytes were injected with 50 nl of cRNA solution and incubated at 17 °C in frog Ringer’s solution containing (in mM): 88 NaCl, 1 KCl, 2.4 NaHCO 3 , 0.3 Ca(NO 3 ) 2 , 0.41 CaCl 2 and 0.82 MgSO 4 , pH7.6 with 0.1% penicillin–streptomycin solution (Sigma-Aldrich). The amount of injected cRNAs of KCNQ1 and KCNE1 were 10 and 1 ng for each oocyte. Two to 4 days after cRNA injection, K + currents were recorded under two-electrode voltage clamp using an amplifier (OC725C; Warner Instruments) and pClamp10 software (Molecular Devices). Data from the amplifier were digitized at 1 kHz through Digidata1440 (Molecular Devices) and filtered at 100 Hz by pClamp10. The microelectrodes were drawn from borosilicate glass capillaries (World Precision Instruments) to a resistance of 0.2–0.5 MΩ when filled with 3 M K-acetate and 10 mM KCl. The bath solution contained (in mM): 96 NaCl, 2 KCl, 1.8 CaCl 2 , 1 MgCl 2 and 5 HEPES, pH 7.2. Oocytes were held at −90 mV, stepped up to various potentials for 2 s (without KCNE1) or 20 s (with KCNE1), and subsequently to −30 mV to record tail currents for conductance–voltage ( G – V ) relationships. All experiments were performed at room temperature (24±2 °C). Animal experiments were approved by the Animal Care Committee of the National Institute for Physiological Sciences and conformed to the guidelines. Analysis of voltage dependence G – V relationships were taken from tail current amplitude at −30 mV. Tail currents were fitted using pClamp10 software to a two-state Boltzmann equation: where G max and G min are the maximum and minimum tail current amplitudes, z is the effective charge, V 1/2 is the half-activation voltage, T is the temperature in degrees Kelvin, F is Faraday’s constant and R is the Boltzmann constant. G / G max , which is normalized tail current amplitude, was plotted against membrane potential for presentation of the G–V relationships. Voltage clamp fluorometry For VCF, defolliculated Xenopus oocytes were injected with 10–25 ng of KCNQ1 cRNA with 1 ng of KCNE1 cRNA. Oocytes were stored at 17 °C in the frog Ringer’s solution for 3–7 days after injection and labelled for 20–30 min with 100 μM Alexa488 maleimide (Life Technologies) in high K + solution (in mM; 98 KCl, 1.8 CaCl 2 , 1 MgCl 2 , 5 Hepes, pH7.2 with NaOH) on ice [34] . Oocytes were placed in a recording chamber with animal pole up. Voltage clamp was performed as described above. A volume of 100 μM LaCl 3 was added only when the voltage went to hyperpolarized potential to block the hyperpolarization-activated endogenous current [34] . Fluorescence recordings were performed with an Olympus fluorescence macrozoom microscope MVX10 through a × 2 objective (MVPLAPO 2XC; NA=0.5; Olympus) and GFP filter cube (U-MGFPHQ/XL; Olympus), with a xenon lamp as the light source. The top of the oocyte could be zoomed by up to × 6.3 magnification with × 2 magnification changer (MVX-CA2X; Olympus); therefore, the total maximum magnification was × 25.2 with the × 2 objective. Fluorescence signals were obtained by a photomultiplier (H10722-110; Hamamatsu Photonics) and digitized at 1 kHz thorough Digidata1440, filtered at 100 Hz and recorded using pClamp10 simultaneously with ionic currents. Oocytes were depolarized from the holding potential of −100 or −80 mV to between −80 or −160 to +80 mV for 2 s with 10-s intervals. To improve signal-to-noise ratio, VCF was repeated five times for each sample, and averaged data were used for presentation and analysis. The shutter for the excitation was open during the recording; therefore, a continuous decrease of fluorescence due to photobleaching was observed. From the base line levels of the initial 500 ms before test pulses of the first and the final traces, we calculated a bleaching rate for each experiment, which usually ranged between 0.01–0.05% per second with 12% ND filter. We then compensated the fluorescence traces by subtracting the expected bleached component calculated from the trace’s own bleaching rate ( R ), assuming the fluorescence was linearly decreased. Arithmetic operations were performed with Clampfit software from pClamp10. where [time] is the time value of the point given by Clampfit. We then normalized the current by setting each baseline level to be 1. Analysis of the VCF Time constants for fluorescence rise and ionic current activation were obtained by a fitting using Igor Pro (Wave Matrices). At lower membrane potential (−40 mV or lower), both the fluorescence and ionic current were generally fitted with a single exponential function while they were fitted with a double exponential function at −20 mV or higher membrane potential. For the slow components, the number of experiments is fewer than those for the fast time constants because sometimes, the fluorescence rise could not be fitted with a double exponential function even at a membrane potential higher than −20 mV. In that case, the traces were fitted with a single exponential function and the obtained time constant was categorized as ‘fast’. Especially for WT without KCNE1, only one out of four traces could be fitted with a double exponential function. This is the reason why the plots of the slower time constant ( Fig. 4b ) and the ratio of fast and slow component ( Fig. 4c ) has no error bar. Structural data presentation Structural data were presented using PyMOL software (DeLano Scientific). Statistical analysis The data were expressed as mean±s.e.m. Differences between means were evaluated using Dunnett’s test or Tukey–Kramer test. Values of P <0.05 were considered significant. *, **, *** denote values of P <0.05, 0.01 and 0.001, respectively. How to cite this article : Nakajo, K. et al . Steric hindrance between S4 and S5 of the KCNQ1/KCNE1 channel hampers pore opening. Nat. Commun. 5:4100 doi: 10.1038/ncomms5100 (2014).